The delusive accuracy of global irrigation water withdrawal estimates 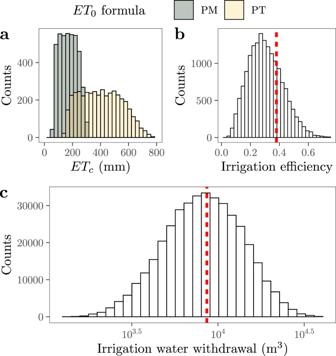Fig. 1: Examples of the ambiguities embedded in the calculation of global irrigation water withdrawals4. aUncertainties in the estimation of the crop evapotranspiration (ETc). PM and PT stand for the Penman–Monteith and the Priestley–Taylor equation, respectively. Data is retrieved from Nichols et al.11. We describe the uncertainty inkcwith the values reported for salt cedar for May4.bDistribution of the irrigation efficiency of China after propagating uncertainties. The red, dashed line marks the efficiency value used by some large-scale models12.cDistribution of the water withdrawn to irrigate wheat in a specific grid cell of the Uvalde County, TX, USA (lon = −99.7083, lat = 29.4583), January 6–7, 2007. All uncertainties in the calculation of IWW are considered4. The red, vertical line is the estimate produced when the uncertain parameters used in the calculation of IWW are characterized with point estimates (e.g., mean values). The estimation of IWW via large-scale models generally follows the relationship between crop yields and water requirement outlined by agronomists and irrigation engineers in the 1950–1960s. In their most simplified form, simulations require data on the extent of irrigation, crop evapotranspiration, precipitation, and irrigation efficiency. Spatially explicit IWW estimates are computed in every grid cell at a given time step and regional, national and global estimates are produced by adding up values at the grid cell level. None of the relevant parameters can be characterized with precise values. Firstly, the extent of irrigated areas is unknown. There are at least four maps of global irrigated areas based on official statistics and remote sensing imagery, and the values they specify differ significantly [3] . For the same grid cell, the reported irrigated area can extend over 30 ha or over 8000 ha depending on the map used [4] . At the national level, the irrigated area may vary by a factor of two or more. This also applies to top-ranking countries in irrigation water consumption such as China and India, whose irrigated areas range between 43–74 and 15–88 Mha respectively. If we assume an approximately linear relation between irrigated areas and IWW [5] , the IWW for China and India can, respectively, be up to two and six times larger or smaller depending upon the map selected. A similar situation occurs with the crop evapotranspiration ET c , which is calculated from the evapotranspiration of a reference crop ET 0 and a crop-specific coefficient k c . There are approximately 40 equations available to compute ET 0 [6] and no agreement as to which one works best in a given context. Since ET 0 is a modeled variable its value cannot be validated against any measurement at the scale required, which in turn hinders the appraisal of its accuracy even under “perfect” input data [7] . The crop coefficient k c is also uncertain as it depends on the crop and its growth stage, but can differ also across individuals and growing conditions. If basic uncertainties in ET 0 and in k c are simultaneously propagated into the estimation of ET c , the resulting crop evapotranspiration values may vary considerably. This is shown in Fig. 1 a for Tamarix ramosissima (salt cedar) in New Mexico (USA), whose potential evapotranspiration in May might be anywhere between 60 and 800 mm. Fig. 1: Examples of the ambiguities embedded in the calculation of global irrigation water withdrawals [4] . a Uncertainties in the estimation of the crop evapotranspiration (ET c ). PM and PT stand for the Penman–Monteith and the Priestley–Taylor equation, respectively. Data is retrieved from Nichols et al. [11] . We describe the uncertainty in k c with the values reported for salt cedar for May [4] . b Distribution of the irrigation efficiency of China after propagating uncertainties. The red, dashed line marks the efficiency value used by some large-scale models [12] . c Distribution of the water withdrawn to irrigate wheat in a specific grid cell of the Uvalde County, TX, USA (lon = −99.7083, lat = 29.4583), January 6–7, 2007. All uncertainties in the calculation of IWW are considered [4] . The red, vertical line is the estimate produced when the uncertain parameters used in the calculation of IWW are characterized with point estimates (e.g., mean values). Full size image At a first approximation, crop irrigation water requirements can be estimated as the difference between the crop evapotranspiration and the effective precipitation. The uncertainty inherent in rainfall occurrence and its effectiveness already hinders knowing how much irrigation water may be needed to ensure the development of the crop [8] . And precipitation datasets are prone to ambiguities due to sparsity in the gauge network, the modeling approach, the specific instruments of satellites or the algorithms used to merge data. Their reported annual precipitation estimates over global land can vary by ±100 mm [9] . Finally, irrigation efficiency is the ratio of the water consumed by the crop to that diverted from the water source to the field. When no water is wasted, irrigation efficiency equals 1. Irrigation engineers assume that efficiencies are mainly defined by the irrigation hardware, with surface, sprinkler and micro-irrigation displaying non-overlapping, increasingly higher irrigation efficiencies. These categories comply with a technology-oriented mindset that disconnects irrigation technologies from their social context while rendering farmers as irrelevant actors in managing irrigation agriculture. Large-scale models sanction this perspective and link countries and/or regions with sharp irrigation efficiency point-estimates that are at odds with the variability of empirically determined efficiencies [10] . Note how the irrigation efficiency of 0.38 used for China by large-scale models turns into a range spanning 0.04–0.77 once basic uncertainties are accounted for [4] (Fig. 1 b). This means that IWW estimates for China can be up to 10 times higher and down to two times lower than current values by simply using an alternative yet equally reasonable irrigation efficiency value. The simulation of IWW in large-scale models does not consider these uncertainties. Each model typically runs under one irrigated area map, one crop evapotranspiration equation, one precipitation dataset and a fixed irrigation efficiency value per country or region. Parameters are described with point-estimates rather than with probability distributions. This means that the resulting IWW estimates are strongly conditioned by the choices made during the model design and are unreliable. We illustrate our point in Fig. 1 c, where we compare the IWW values produced using the approach of large-scale models (point-estimates) with those produced when uncertainties are propagated with a global uncertainty and sensitivity analysis. We focus on a grid cell in Uvalde (Texas, USA) given the availability of data for all parameters and the strong reliance of the region on irrigation to produce vegetables and grains. We calculate IWW for wheat for just a single day in January [4] . With point-estimates (e.g., mean values) characterizing each parameter, IWW equal 8600 m 3 . With a thorough propagation of uncertainties, IWW estimates range between 1400 and 40,000 m 3 , thus spanning more than one order of magnitude. It is important to stress that this uncertainty affects only one day and one of the several hundred thousand grid cells included in large-scale models. Should this analysis be repeated in all the grid cells and the results added up to compute yearly national and global IWW estimates, the resulting uncertainty ranges in IWW are likely to be of the utmost importance. Simply put, current IWW estimates present us with a mirage of accuracy. The computation of IWW estimates currently ignores uncertainties. This constitutes a neglect of relevant available evidence and a dangerous complacency in the achievement of the SDGs connected with irrigated agriculture. In our example (Fig. 1 c), the use of county-level IWW point-estimates (the red bar) could grossly misdirect irrigation strategies to manage water stress (SDG 6.4.2) because its account of the water required by crops neglects plausible variations and potential extreme values. Omitting uncertainties can also make water managers issue fixed water licenses that do not reflect varying water availability and water requirements’ evolution over time [13] . By the time the error is amended, the social–ecological damage may have become irreversible. We suggest three corrective measures: First, assume that uncertainties may not disappear. An excess of artificial certainty prematurely locks in a solution, leaving decision makers blind to possible, eventually better, policy alternatives [14] . IWW models are currently pursuing hyperresolution representations (the production of estimates at a 1 km resolution and/or every 1–3 h) to produce more accurate estimates [15] . But this path is unlikely to deliver: greater model detail tends to produce model indeterminacy when uncertainties are thoroughly examined [16] . Increasingly complex models are also likely to usher in more uncertainties due to error propagation and the emergence of new phenomena. This is well known by the climate change community after more than 30 years collecting data on temperature sensitivity to changes in CO 2 atmospheric concentration, leading to increasing intervals [10] , [17] . We argue that uncertainties result from the way we produce knowledge and cannot be banished from science [18] . Rather than trying to eliminate them with more computational power, we might make better progress by developing methodological and conceptual tools to expose them, assimilate them and make them actionable in the real world. Second, utilize computational power to accurately quantify uncertainties. Uncertainties should no longer be appraised with one-at-a-time (OAT) methods and model ensemble designs [19] . OAT cannot explore the uncertainty space of multidimensional models and completely misses the influence of interactions [20] . Model ensembles do not sample all model formulations and are unsystematic [21] . Rather than sustaining the quest towards ever-realistic models, computational power should be invested in stringent global uncertainty and sensitivity analysis. Apart from Monte-Carlo approaches (Fig. 1 c), cost-effective methods such as cheaper-to-run emulators or convergence monitoring allow a much better exploration of the uncertain space than OAT or model ensembles [22] . The outcome will be IWW estimates whose range better matches our knowledge gaps. This is a significant step ahead even if the resulting intervals are too large to be useful for policy-making: in this case, it will suggest that we should leave models aside and turn towards tools better suited to guide policies under irreducible uncertainties, such as deliberative/participative approaches [23] , quantitative storytelling [24] or robust decision making [25] . Finally, expose assumptions and value-ladenness. By formalizing irrigation withdrawals as universal equations guided by engineering goals, large-scale irrigation models exclude the values, interests and behaviors of those with the highest stakes in the issue: farmers and irrigators. For instance, the underlying premise that irrigation should optimize crop production and water use is at odds with the goals of traditional irrigators, whose farming practices result in crop diversity rather than maximum productivity [26] . Such differences can amplify the mismatch between what is modeled and the real-world and can eventually lead to a scenario where the model, and not the system of interest, ends up being the object of management. An example is the Chesapeake Bay Program watershed model, whose output was used by regulators to claim that their policies improved the water quality of the main stem of the Bay despite real water monitoring analysis showing no proof of improvement [27] . These biases may be prevented by conducting action-research and involving local knowledge holders in the modeling process. In Pickering, a British town hit by several floods between 1999 and 2007, the participation of stakeholders helped identify upstream storage processes as a critical element initially overlooked by the designers of the flood risk model used to guide decision-making [23] . The result was a model with a higher legitimacy and honed to the social–environmental particularities of Pickering. Local experts with access to national and river basin-scale water accounts may also help assess the accuracy of IWW at the local level, thus enhancing the credibility of subsequent estimates. Large-scale hydrological models should embrace uncertainties lest they become irrelevant tools for future water management. Supplementary information, including the code to replicate our results, is available in Puy et al. [4] and in https://github.com/arnaldpuy/ghm_auditing .